Sensitive response of the Greenland Ice Sheet to surface melt drainage over a soft bed The dynamic response of the Greenland Ice Sheet (GrIS) depends on feedbacks between surface meltwater delivery to the subglacial environment and ice flow. Recent work has highlighted an important role of hydrological processes in regulating the ice flow, but models have so far overlooked the mechanical effect of soft basal sediment. Here we use a three-dimensional model to investigate hydrological controls on a GrIS soft-bedded region. Our results demonstrate that weakening and strengthening of subglacial sediment, associated with the seasonal delivery of surface meltwater to the bed, modulates ice flow consistent with observations. We propose that sedimentary control on ice flow is a viable alternative to existing models of evolving hydrological systems, and find a strong link between the annual flow stability, and the frequency of high meltwater discharge events. Consequently, the observed GrIS resilience to enhanced melt could be compromised if runoff variability increases further with future climate warming. Variations in the Greenland Ice Sheet (GrIS) flow have been observed on timescales varying from hours to years [1] , [2] , [3] , [4] , [5] , [6] , [7] . In particular, the sudden delivery of surface meltwater to the bed during supraglacial lake (SGL) drainage events drive pronounced although short-lived, accelerations in flow [1] , [2] . Water stored in SGLs is known to attain the bed through hydro-fracturing [1] , [8] , causing rapid and high-magnitude perturbations to the basal environment, where the large and sudden influx of water likely overwhelms the existing drainage system [1] , [2] , [3] , [4] , [5] , [6] , [7] , increasing basal water pressure and reducing ice–bed coupling. Surface melt and storage in SGLs occurred at higher elevations during recent warm summers, and are expected to expand inland as climate warms [9] , [10] , [11] , but it remains unclear how this will affect ice flow. Interpretation of field observations is complex, with some studies suggesting that more melt will increase annual flow [12] , [13] , [14] while others suggest the opposite [15] , [16] , [17] , [18] . Current theoretical understanding of GrIS basal hydrology calls on the evolution of the subglacial drainage system from low to high hydraulic efficiency, to accommodate for melt supply variability over the ablation season [19] , [20] , [21] , although limited direct observations of the basal environment do not fully verify this model [22] , [23] , [24] . Moreover, the representation of an evolving subglacial drainage system in numerical models is challenging, and currently necessitates major simplifications such as reduced spatial dimensions [23] , [25] , [26] , [27] , [28] , application on idealized domains [25] , [29] or disregarding feedbacks on ice flow [30] . Significantly, these dynamic processes are yet to be realistically incorporated into studies aiming to forecast future sea-level rise [31] , [32] , [33] . In addition, by focusing explicitly on the character of the hydrological system, previous work has inherently assumed that the ice–bed interface consists of hard bedrock. However, thick subglacial sediments have been observed [34] , [35] and furthermore are known to exert first-order control on flow in other glaciated regions [36] , [37] , [38] , [39] , [40] , [41] . To date, theoretical considerations on the implications of a soft sedimentary bed on GrIS dynamics are only starting to emerge [42] , but have never been implemented and tested in modelling studies. Here we use surface melt, runoff and SGL discharge across the wider Russell Glacier (RG) catchment during summer 2010 (refs 10 , 43 ), to drive the higher-order three-dimensional Community Ice Sheet Model (CISM), coupled with models of subglacial sediment and basal hydrology. We find that delivery of surface meltwater to the bed can induce the observed seasonal ice flow variability through the hydro-mechanical response of soft basal sediments. We identify meltwater stored in SGLs as the primary forcing of GrIS seasonal ice flow, and we show that SGL drainage over a soft bed can display a stabilizing effect similar to that so far explained in existing hydrological models [19] , [20] , [21] . This apparent ice sheet stability is, however, reduced when the effect of increasing runoff variability is included in our soft bed model. A relationship between the frequency of high surface meltwater discharge events in summer and annual ice flow stability is uncovered in this study, and points to GrIS as being more vulnerable to climate warming than projected [44] . Ice-water-sediment interactions beneath RG The physical properties in the subglacial sediment model integrates recent geophysical observations, revealing where available that RG is underlain by a porous, mechanically weak sediment [34] , [35] , of similar character to tills produced by glaciers in Canada and Svalbard [37] , [45] (see Methods). The subglacial sediment model was coupled to a hydrological model, which has previously been used to calculate the routing and fluxes of water associated with the episodic drainage of subglacial lakes in Antarctica [46] , and is well suited for analysis of SGL drainage events. The explicit inclusion of interacting models of subglacial sediment and water is new, yet consistent with the extremely high suspended sediment loads observed in proglacial streams draining RG catchment [47] , [48] . The latter equates to bulk catchment erosion rates of 4.8 mm a −1 (ref. 48 ), which is far greater than other rates estimated for regions where glaciers override a hard crystalline rock (0.004–0.1 mm a −1 , refs 49 , 50 ). Current understanding of SGL dynamics suggest that a rapid, high-magnitude influx of water to the bed (considering peak fluxes as high as 5,000 m 3 s −1 , ref. 10 ) cannot be instantaneously accommodated by expansion of a channelized basal drainage system [51] . Rather, the accelerated flow observed in late summer, when an efficient drainage system had already developed [12] , [28] , [51] , points to subglacial evacuation of water in a high-pressure system [5] , [30] . Here, we assume that meltwater delivered to the bed is transported down the hydraulic potential surface in an efficient basal water system, which coexists and interacts with a hydraulically inefficient subglacial sediment layer. The physics controlling the rate of water infiltrating the sediment layer is likely complex, but with a paucity of data to constrain this interaction, we use a simple parameterization in which basal water is transferred into the underlying sediment in proportion to the magnitude of the horizontal water flux associated with the hydrological forcing (See Methods). This perturbation induces excess pore pressure and vertical hydraulic gradients, and thus flow of water within the sediment, which increases its porosity accordingly. This causes sediment shear strength to drop, along with basal traction and resistance to ice flow (equation (1)). The expansion of sediment pore space is represented in our model through compressibility, a well-established material property, which has been determined for a variety of subglacial tills [37] , [52] . In this manner, we assessed the time-varying hydrological impact of seasonal meltwater delivery on subglacial sediment shear strength, thereby defining patterns of basal traction across the model domain at a horizontal resolution of 1 km (see Methods). The model was initialized by performing a data inversion on a composite image of the winter 2010 observed velocity ( Fig. 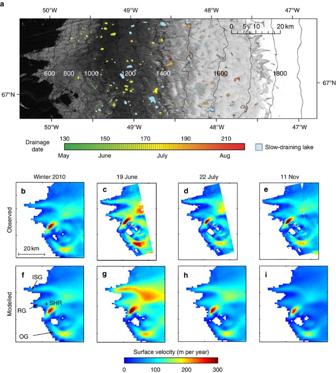Figure 1: Supraglacial lakes and seasonal ice flow in the Russell Glacier catchment. (a) Colour-coded summer 2010 lake-drainage map, with elevation contours (m). (b) Composite winter 2010 observed velocity map (m per year). (c–e) Velocity maps (m per year) derived from TerraSAR-X satellite data, showing the average velocity over 11-day periods centred over the date indicated above each panel. (f) Modelled initial ice flow for winter 2010 (m per year). (g–i) Modelled ice flow (m per year) averaged over the same 11-day periods used to generate TerraSAR-X velocity maps as shown inc–e. The locations of Russell Glacier (RG), Isunngata Sermia Glacier (ISG), Orkendalen Glacier (OG) and SHR site are indicated inf. 1 ; Table 1 , see also Methods). We then performed a series of forward experiments for a 6-month period starting on the 15 May 2010 (Methods). First, we investigated the impact of SGL drainage events by forcing the model with the 2010 record of drained SGL volumes [10] ( Fig. 1a ; Supplementary Movie 1 ). Second, we examined the effect of the runoff produced daily in each SGL sub-catchment for that same year [43] . Third, we tested the possibility that ice flow responds to hydrological perturbations defined by the variability in runoff together with SGL drainage events ( Supplementary Movie 2 ). Figure 1: Supraglacial lakes and seasonal ice flow in the Russell Glacier catchment. ( a ) Colour-coded summer 2010 lake-drainage map, with elevation contours (m). ( b ) Composite winter 2010 observed velocity map (m per year). ( c – e ) Velocity maps (m per year) derived from TerraSAR-X satellite data, showing the average velocity over 11-day periods centred over the date indicated above each panel. ( f ) Modelled initial ice flow for winter 2010 (m per year). ( g – i ) Modelled ice flow (m per year) averaged over the same 11-day periods used to generate TerraSAR-X velocity maps as shown in c – e . The locations of Russell Glacier (RG), Isunngata Sermia Glacier (ISG), Orkendalen Glacier (OG) and SHR site are indicated in f . Full size image Table 1 Comparison of remotely sensed data and model output. Full size table Seasonal ice flow driven by observed SGL drainage The 2010 record of SGL drainage volumes was first used to drive the model. Patterns of surface velocity derived from TerraSAR-X satellite image pairs acquired with 11-day separation and centred on 19 June, 22 July and 11 November [53] , [54] are shown in Fig. 1 together with maps of modelled surface velocity averaged over the exact same periods. Flow acceleration, both observed and modelled, is most apparent on 19 June, ~30 km from the margin of RG, and for Orkendalen Glacier, south of RG ( Fig. 1 ). On 22 July, modelled and observed surface velocities have declined substantially, and by 11 November, both have approached the previous winter mean. Modelled seasonal flow evolution is in overall good agreement with the TerraSAR-X velocity snapshots, with net errors of 10% and correlation coefficients of 0.79–0.94 ( Table 1 ). To assess model efficacy and its ability to capture the dynamic events observed, continuous model output was compared with daily mean surface velocity measured by a Global Positioning System (GPS) receiver at the SHR site ( Fig. 1 ), ~15 km from the margin of RG ( Fig. 2a ). All the main velocity features at SHR are captured in the model; throughout June, July and August, modelled mean daily velocity at SHR was generally well estimated (within 16%), with a good correlation to observed values ( r 2 =0.83, Supplementary Table 1 ). On 10 June, modelled velocity at SHR attained a maximum of 326 m per year, within 6% of that measured by GPS. Likewise, on 25 June modelled velocity peaked at 248 m per year, within 15% of that observed. Noteworthy however, is that the model did not initially reproduce the first ‘spring-event’ acceleration in late May, as fluxes calculated from SGL drainage events were insufficient to perturb subglacial conditions at SHR ( Supplementary Fig. 1 ). To reproduce this first spring event, the lake volume loss on 24–27 May needed to be three times those shown in Fig. 2b . The model may be unable to sufficiently respond to spring-event stimuli possibly because the ice flow may be more sensitive to water input in the lower ablation zone early in the melt season, when the basal system is not yet fully developed [12] , [51] . Another plausible explanation is that basal meltwater produced in situ by frictional and geothermal heating accumulates at the bed over the course of winter and is released together with the first SGL drainage events. 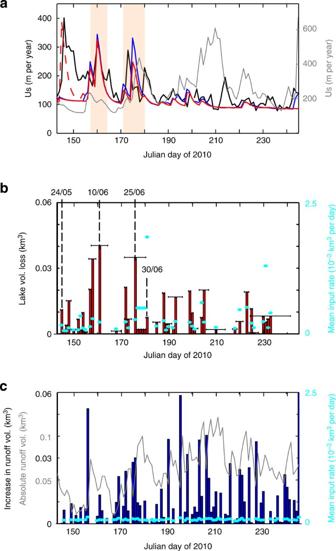Figure 2: Modelled versus observed daily mean ice flow speeds at site SHR and daily water forcing estimated for RG catchment. (a) Timeseries of observed mean daily velocity acquired with Global Positioning System at the SHR site (black), and comparison with model output at the same location, when forced with SGL-only volumes (red), with SGL volumes plus runoff rates (blue) and with absolute runoff volumes (grey, RHS scale). The speed-up event on 24–27 May is reproduced assuming a threefold increase in SGL volume loss (red dashed line). This can be explained, as in reality, the ice flow may be more sensitive to water input early in the season, when the basal water system is not yet fully developed. Alternately, the observed ice flow may have responded to SGL water loss combined with the basal meltwater produced over winter and released early in the ablation season. The shaded red zone corresponds to uncertainties in observing the timing of SGL drainage on 10 June and 25 June, due to cloud cover. (b) SGL volume loss data used to drive the model. For periods of time where no satellite data were available (horizontal bars), the timing of drainage is centred over that period10. (c) Daily runoff rates (blue bars), calculated from the total runoff volume estimated for 2010 (ref.43) (grey line). The daily mean water input rates (RHS scale, cyan dots inb,c) are highest for SGL volume loss. Figure 2: Modelled versus observed daily mean ice flow speeds at site SHR and daily water forcing estimated for RG catchment. ( a ) Timeseries of observed mean daily velocity acquired with Global Positioning System at the SHR site (black), and comparison with model output at the same location, when forced with SGL-only volumes (red), with SGL volumes plus runoff rates (blue) and with absolute runoff volumes (grey, RHS scale). The speed-up event on 24–27 May is reproduced assuming a threefold increase in SGL volume loss (red dashed line). This can be explained, as in reality, the ice flow may be more sensitive to water input early in the season, when the basal water system is not yet fully developed. Alternately, the observed ice flow may have responded to SGL water loss combined with the basal meltwater produced over winter and released early in the ablation season. The shaded red zone corresponds to uncertainties in observing the timing of SGL drainage on 10 June and 25 June, due to cloud cover. ( b ) SGL volume loss data used to drive the model. For periods of time where no satellite data were available (horizontal bars), the timing of drainage is centred over that period [10] . ( c ) Daily runoff rates (blue bars), calculated from the total runoff volume estimated for 2010 (ref. 43 ) (grey line). The daily mean water input rates (RHS scale, cyan dots in b , c ) are highest for SGL volume loss. Full size image Seasonal ice flow driven by observed SGL drainage and runoff We isolated and tested the extent to which SGL drainage controls seasonal ice flow by performing experiments in which the model was driven by local runoff production delivered to the bed in each SGL sub-catchment (see Methods). Using total daily runoff volumes [43] , we found that modelled ice flow was fastest in late July ( Fig. 2a ; Supplementary Figs 2 and 3 ), an outcome inconsistent with the relatively slow flow observed at this time ( Figs 1 and 2a ) [12] , [54] . This discrepancy is not surprising since both theory and observations demonstrate that it is the variability rather than the absolute volume of meltwater delivery to the bed that drives ice flow dynamics [19] , [27] , [28] , [51] , [55] . Indeed, a reduction in the daily variability of surface melt at this peak period of runoff feasibly explains why observed ice flow remained slower from early July and onwards [28] , a reasoning consistent with the existence of an efficient system capable of evacuating large volumes of water. Our total runoff experiment supports this interpretation. The model was unable to reproduce seasonal ice motion when assuming that the sediment layer takes in all of the runoff, which suggests that some of this water is instead integrated in an existing efficient hydrological system. Accordingly, we performed a final suite of experiments in which the model was forced with daily meltwater perturbations, including the estimated daily difference in runoff in addition to the SGL drainage volumes. The underlying assumption for these experiments is that it is the sum of positive daily increases in runoff at each sub-catchment and the SGL volume that collectively represents the net hydrological forcing to which the ice flow responds (equation (7)), and that the remaining quantity of water is routed to the margin without effect (as previously inferred [18] , [19] , [28] , [51] , [55] ). Although the forcing volume of water was over three times greater than in the SGL-only drainage experiments ( Fig. 2c , see Methods), the model was still able to successfully yield the observed flow structure ( Fig. 2a ; Supplementary Figs 2 and 3 ), showing no appreciable difference to the SGL-only runs ( Table 1 ; Supplementary Table 1 ). This limited impact stems from the fact that daily differences in runoff calculated at each lake site (henceforth referred to as runoff rates) were smaller than the typical volume of water contained in lakes observed to drain ( Fig. 2b,c ). These results suggest that the hydrological forcing associated with the runoff variability alone was not capable of inducing a substantial ice flow response in 2010 ( Supplementary Fig. 3 ). Impact of SGL discharge on basal sediment properties In our model, water at the ice–sediment interface travels 20–70 km down glacier in 1 day, an efficient routing that is consistent with SF6 gas tracing experiments that estimate subglacial water velocities from 22 to >86 km per day (ref. 22 ). As water travels down the hydraulic potential surface, it interacts with the hydraulically inefficient subglacial sediment layer below it. On 10 June, modelled water fluxes locally attain 570 m 3 s −1 ( Fig. 3a ) and average 57 m 3 s −1 over a distance of ~65 km. The volume of water entering the sediment was 3.8 × 10 6 m 3 , which is ~10% of the lake water available on that date. The remaining ~90% is routed away by the basal hydrological system. This is consistent with observations, which demonstrate that the majority of water delivered to the bed travels to the ice margin within a few days [10] , [22] , [28] , [43] . Nevertheless, local sediment shear strength and basal traction fell to about a third (~50 kPa) of the pre-discharge value ( Fig. 3c ), as the porosity of the sediment increased with the water intake (equation (1) and Supplementary Fig. 4 ). This led to a substantial (up to 200%) surface flow acceleration in a region considerably larger than that of the local meltwater production and input, and extending as far as the ice sheet’s margin ( Fig. 3b,d ). Furthermore, an equivalent sediment strengthening took place over the following days (12–13 June, Fig. 3e ), as pore-water pressure within the temporarily expanded sediment layer returned to its post-pulse equilibrium driving a net flow deceleration of up to 75% ( Fig. 3f ). 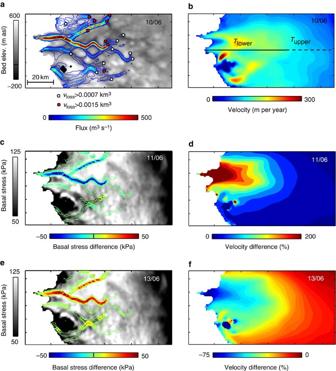Figure 3: Modelled dynamic impact of SGL drainage on 10 June 2010. (a) Bed elevation (m a.s.l., grey scale) overlain with modelled water flux (m3s−1, colour scale) from lakes draining on 10 June (red and white dots,vloss). (b) Modelled (pre-discharge) mean daily velocity on 10 June (m per year). (c) Modelled basal shear stress (kPa, grey scale) overlain with basal stress reduction calculated on 11 June (kPa, colour scale) and (d) associated speedup (%). (e) Modelled basal shear stress (kPa, grey scale) overlain with increase in basal stress calculated on 13 June (kPa, colour scale), relative to that calculated on 11 June, and (f) associated slowdown (%). The location of transects (Tlower,Tupper) used to calculate velocities inFig. 4is shown inb. Figure 3: Modelled dynamic impact of SGL drainage on 10 June 2010. ( a ) Bed elevation (m a.s.l., grey scale) overlain with modelled water flux (m 3 s −1 , colour scale) from lakes draining on 10 June (red and white dots, v loss ). ( b ) Modelled (pre-discharge) mean daily velocity on 10 June (m per year). ( c ) Modelled basal shear stress (kPa, grey scale) overlain with basal stress reduction calculated on 11 June (kPa, colour scale) and ( d ) associated speedup (%). ( e ) Modelled basal shear stress (kPa, grey scale) overlain with increase in basal stress calculated on 13 June (kPa, colour scale), relative to that calculated on 11 June, and ( f ) associated slowdown (%). The location of transects ( T lower , T upper ) used to calculate velocities in Fig. 4 is shown in b . Full size image Sensitivity to surface water inputs In all our experiments ( Supplementary Fig. 3 ), modelled ice flow at the end of the season was slower than that at the start (winter 2009/10). Although this seasonal velocity reduction may be subtle ( Fig. 2a ; Supplementary Fig. 3 ), it is a consistent feature of the model’s sensitivity to surface meltwater delivery to the bed ( Fig. 4 ; Supplementary Fig. 5 ). This modelled self-regulation of ice flow is consistent with recent findings from GPS measurements across the ablation area of RG, revealing that flow enhancement from increased surface melting during warm summers is negated by reduced winter velocities [17] , [18] . To date, the latter has been exclusively attributed to increased effective pressure provided by summer expansion of subglacial channels over a hard bed [19] , [20] , [21] , [28] , [51] . Here, model results provide an alternative explanation for the soft-bed condition. Summer ice flow is greater with higher SGL discharge because higher hydraulic gradients drive a proportionally larger volume of water into the subglacial sediment layer (Methods, equations (2) and (3)). Upon evacuation of surface meltwater, reversed but equally high hydraulic gradients develop and drive water out of the sediment. With sufficiently high gradients, the new state of water pressure equilibrium in the sediment is attained with an overall sediment strengthening compared with its pre-summer state, and therefore lower velocities in autumn. 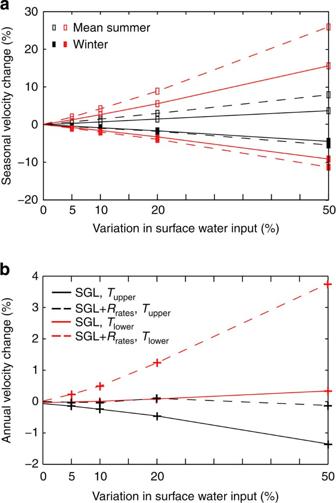Figure 4: Modelled ice flow sensitivity to variation in surface water inputs. Modelled velocity along the transectsTlower(red) andTupper(black), using SGL-only volumes (solid lines) and runoff rates in addition to SGL volumes (dashed lines). SeeFig. 3for transects location. (a) Change (%) in mean summer velocity (open squares) and winter velocity (coloured squares). The latter is assumed to be represented by the end-of-run (15 November) value. (b) Mean annual velocity change (%). Figure 4: Modelled ice flow sensitivity to variation in surface water inputs. Modelled velocity along the transects T lower (red) and T upper (black), using SGL-only volumes (solid lines) and runoff rates in addition to SGL volumes (dashed lines). See Fig. 3 for transects location. ( a ) Change (%) in mean summer velocity (open squares) and winter velocity (coloured squares). The latter is assumed to be represented by the end-of-run (15 November) value. ( b ) Mean annual velocity change (%). Full size image To test the ice sheet sensitivity to enhanced surface melt, the coupled models were used to examine changing ice flow along two transects (shown on Fig. 3b ), to differentiate between the region of significantly enhanced ice flow ( T lower , 0–60 km inland) and that upstream of this limit ( T upper , 60–95 km inland). When SGL-only volumes were increased by up to 50%, the combined effects of faster summer flow (16% for T lower and 4% for T upper ) and reduced winter flow (−9% for T lower and −5% for T upper ) ( Fig. 4a ) translated into relatively constant annually averaged flow along T lower (+0.3%) and a slight decrease (that is, self-regulation) along the upper region ( T upper ~ −1%; Fig. 4b ). Model sensitivity was investigated by also assuming a 50% increase in runoff, which directly leads to an equivalent 50% increase in the runoff rates. Results indicate that summer flow was significantly enhanced (26% for T lower and 8% for T upper ) consistent with observations [13] , [17] , [18] . However, the subsequent winter slowdown (−11% for T lower and −5% for T upper ) was in this case insufficient to offset the summer increase ( Fig. 4a ). Hence, under increased runoff, modelled annual velocities along T lower increased by ~4%, while farther inland, annual flow was no longer stabilized by a negative feedback ( Fig. 4b ). The explanation is apparent from the nature of the two forcing sets. The 2010 SGL drainage record encompasses ~500 discrete high-rate discharge events. The runoff rates record includes >2,500 events, but the majority of these events are of a smaller magnitude compared with SGL drainage ( Fig. 2b,c ). However, under enhanced surface melting the potential for runoff to influence ice dynamics is obvious. With our model, when surface runoff is increased by 50%, a substantial number of distinct runoff rate events, originally too small to have an impact on ice flow, become comparable in magnitude to individual SGL drainage events. As a result of the combined effect of SGL and runoff, subsequent winter slowdown cannot compensate for the discrete summer acceleration events, and hence there is a net positive increase in mean annual flow, modelled well into the ice sheet interior. The modelling presented is the first to quantitatively reproduce the flow evolution at the GrIS margin over a complete ablation season. The model accurately replicates both temporal and spatial characteristics of the observed flow, as a result of changes in basal traction caused by delivery of surface meltwater to a soft-bed ( Supplementary Movies 1 and 2 ). For the 2010 melt season, runoff events had a limited impact on ice flow because individual discharge variability associated with the full-melt record remained significantly lower than that of SGL drainage. Thus, we conclude that SGL drainage events presently exert a primary control on GrIS seasonal ice-flow variability, as has been previously hypothesized [1] , [3] , [5] , [8] . While our study confirms a strong hydrological control on ice flow, it also reveals that this control may occur through its interaction with subglacial sediment and not exclusively from the evolution of hard-bedded drainage system configurations as previously assumed [15] , [19] , [28] , [51] . Our results demonstrate that the effect of water flowing into and out of soft subglacial sediment strongly resembles the anticipated effect of basal drainage system switches, but with significant long-term differences. For the soft-bedded portion of the GrIS, we predict that any future increase in surface melt volumes will lead to faster net summer flow. However, the evolution of the annual velocity appears to depend on the number of high-magnitude discharge events. We find that with SGL drainage-only forcing, the annual ice flow is resilient to enhanced surface melting, even if the SGL drainage increases by up to 50% in volume. This can explain the recently observed stable response to increased summer melting in this region [17] , [18] , [56] . However, if the spatial distribution and frequency of high discharge events increases, for example, due to higher runoff variability as expected in a warming climate [11] , [57] , net annual ice flow is likely to increase, rather than decrease. Similar trends have been found in recent modelling studies examining the longer-term effect of enhanced melt on ice flow [29] , [32] . Further observations and modelling is required to weigh-up the role of evolving subglacial channels versus sediment control on ice flow, in particular in the context of enhanced meltwater delivery to the bed. Direct observations of the subglacial environment are an outstanding requirement to further assess this uncertainty, and to provide accurate constraints on the long-term fate of the GrIS in a warmer climate. Ice sheet model Ice flow response to surface meltwater drainage events was investigated by coupling the higher-order thermodynamic model CISM to a model of subglacial sediment [40] , as well as a model of subglacial hydrology [46] . The ice thickness evolves according to the continuity equation; conservation of energy is expressed through the advective-diffusive heat equation. The coupling between the ice flow and sediment models is done via the determination of the porosity-controlled basal shear strength at the top of the modelled sediment layer. The latter is used to calculate the basal stress in the force balance equation of CISM, assuming a plastic yield stress basal boundary condition (see ref. 40 for full details on the ice-flow model, and its coupling to the subglacial sediment model). Basal sediment model For a shearing soil, the sediment strength ( τ f ) and its porosity ( n ) are both independently related to the sediment-effective pressure ( N ), such that τ f ∝ N and n ∝ log( N ) [37] , [38] , [58] . Using these two relationships, one can calculate the sediment strength as a function of sediment void ratio ( e , a quantity related to the porosity as n = e /(1+ e )) (equation (3c) in ref. 38 , see refs 37 , 38 for full details): where e o is the void ratio value at the reference value of effective normal stress N o , C is the sediment compression index and φ is the sediment internal friction angle. Values of e o , N o , C , φ are set to those of Trapridge till [37] , which are also similar to parameters established for till beneath glaciers in Svalbard [45] ( Supplementary Table 2 ). To solve equation (1), we calculate changes in sediment porosity throughout the layer ( Supplementary Fig. 4 ) from mass conservation, dictated by Darcian vertical water flows within it ( v w , equation (2) below). The latter are driven by hydraulic gradients, here expressed with the excess, rather than total, water pressure [59] , [60] . Note that the total water pressure is such that P w = P h + u , where P h is the hydrostatic pressure and u is the excess pore pressure: where u is the excess pore-water pressure in the sediment (Pa), K h is the sediment hydraulic conductivity (m s −1 ), ρ w is the water density (kg m −3 ), g is the gravitational acceleration (m s −2 ) and z is the vertical coordinate (m). Lateral water fluxes in the sediment layer are ignored [61] . We further note that without an explicit representation of the channelized subglacial drainage system, we cannot account for variation in effective pressure related to such a system. The order of magnitude difference between our model resolution (1 km) and the anticipated channels’ diameter (a few metres across) supports this model simplification. Finally, the excess pore pressure distribution in the sediment layer is obtained from [59] : where, t is the time (s), C v is the sediment diffusivity (m 2 s −1 ), is the initial domain-averaged sliding velocity (m s −1 ), scaled with a factor f to facilitate vertical advection of water through the sediment (modified from previous work [60] ). Values of physical constants and model parameters for all equations are summarized in Supplementary Table 2 . Basal water system model The horizontal water fluxes ( ψ , m 3 s −1 ) associated with water discharge and the corresponding basal water thicknesses are calculated at each time step using a steady-state directional routing algorithm. The flux is distributed among eight neighbouring grid cells, where cells with lower hydraulic potential receive a fraction of the outflow, depending on the local slope of the hydraulic potential surface ( h , m) [46] , [62] . where ψ in is the incoming flux, i is the index of the current grid cell, m is the running index of adjacent grid cells, k is the number of cells with lower hydraulic potentials and s is the distance to the adjacent cell. In line with other work on subglacial water flow in a distributed system [62] , we assume the flow to be laminar, noting that this assumption would not apply to flow in channelized systems (not explicitly included here). As derived elsewhere [62] , the water thickness ( d wat , m) of a laminar flow in a distributed thin water film is calculated using: where μ is the water viscosity, and θ is the hydraulic potential (Pa). The latter is here defined as: where Z bed is the bed elevation (m), H is the ice thickness (m), ρ i is the ice density (kg m −3 ) and N is the effective pressure (Pa), here calculated from the sediment strength at the top of the sediment layer. Boundary conditions in the sediment layer When a large volume of water is transiently delivered to the bed, excess pore-water pressure and vertical hydraulic gradients drive water flow downwards and into the sediment (equation (3)). The hydraulic gradient at the ice–sediment interface is calculated from equation (2) [61] , with the rate of water entering the sediment layer ( , m s −1 ) estimated as follow: where V melt is the melt rate (m s −1 ) calculated from the basal heat budget, V hydro is the distributed water thickness available at the ice bed ( d wat ) adjusted per time unit (m s −1 ), ψ max (m 3 s −1 ) and the dimensionless exponent α are two empirical constants. We prescribed a 5-m-thick sediment layer, with a no-flux bottom boundary condition. Whereas prescribing a thicker sediment layer had little impact on model output ( Supplementary Fig. 5 ), we have not investigated the potential effect of an uneven and patchy distribution of sediment, an experiment beyond the scope of this study. We note that, over the course of summer, only the top 2 m of the modelled sediment layer are affected by water inflow ( Supplementary Fig. 4 ), consistent with observations [35] . Model initialization We used high-resolution surface and subglacial topography, which exert primary control on the subglacial distribution and flow of water [5] , [63] . The geometry is prescribed using a 2008 SPOT surface digital elevation model (DEM) at 40-m resolution [64] , and a 500-m bed DEM produced from ice surface and thickness measurements from NASA’s Operation IceBridge supplemented by additional radio-echo sounding data acquired by ground-based field campaigns. Each was resampled at the model resolution of 1 km. The initial conditions of flow were obtained by performing a model inversion, using the composite image of the winter 2010 observed velocity ( Fig. 1b ), and following an iterative technique where the basal traction coefficients are determined so that the modelled surface velocities converge towards those observed [65] . Besides setting the initial velocity field, the model inversion provides a steady-state temperature field (assuming temperature at the pressure-melting point at the ice base) and the initial spatial distribution of basal traction. The initial sediment void ratio (porosity) is obtained by solving equation (1), assuming that the sediment shear strength is equal to the initial basal traction derived from model inversion. The resulting initial porosity values range from 22 to 32%, in agreement with values inferred for RG from seismic surveys [35] . Surface water forcing The model was forced using three representations of surface melt, as shown on Fig. 2b,c (results for sensitivity tests on the type of surface melt forcing are shown in Supplementary Figs 2 and 3 ): 1 First, we used a record of drained SGL volumes, totalling 0.43 km 3 ( Fig. 2b ). The timing and location of SGL drainage was derived from daily MODIS imagery, and lake volumes were estimated using a depth–reflectance relationship. Full details on the SGL record used here are available in ref. 10 . 2 We then ran the model using absolute runoff volumes calculated for 2010 ( [43] ) ( Fig. 2c , grey line), totalling 6.58 km 3 . The daily, distributed runoff volumes were estimated with a surface energy balance model using automatic weather station measurements and MODIS-derived albedo as inputs [43] . Daily runoff for each lake catchment was then derived using the ArcGIS hydrology toolkit and a 30-m DEM as input. 3 Finally, we used the runoff record to specify the daily variation, allowing us to examine the effect of runoff variability rather than its absolute volume ( Fig. 2c ). These ‘runoff rates’ were defined as positive when the daily melt increased compared with the previous day, and were set to zero when daily melt decreased. The runoff rates, used to force the model, represent a total water volume of 1.03 km 3 . This experiment is equivalent to assuming that 5.55 km 3 of the full runoff (6.58 km 3 ) is routed along the bed with no further effect on ice flow. The volume defined by runoff rates (1.03 km 3 ) comprises water volumes, which cannot be accommodated by an existing hydrological system. These volumes were inserted at lake locations, and allowed to interact with the subglacial sediment (equation (7)) while being routed in the basal water system (equation (4)). Testing the model We tested three particular aspects of the model setup: 1 We tuned the model by testing a range of parameter values for equation (7). Values of ψ max ranged from 400 to 700 m 3 s −1 . Values of the dimensionless exponent α ranged from 1 to 2 ( Supplementary Table 2 ). The results discussed in the main article were obtained by setting α to 2, and ψ max to 500 m 3 s −1 , while results using alternate values are shown in Supplementary Fig. 3 . 2 A uniform application of equation (7) in both space and time is chosen for simplicity. This may limit the model’s ability to reproduce spring events, as explained in the main article. Similarly, for Isungata Sermia Glacier (in Fig. 1 ), GPS observations show a much lower amplitude of summer flow variations here compared with RG and glaciers farther south ( Supplementary Fig. 6 ), despite generally high water discharge and velocity. The latter may be connected in that persistently high fluxes of subglacial water at Isungata Sermia Glacier may render this glacier less sensitive to surface water inputs due to a large and well-developed subglacial drainage system close to the margin [23] . 3 Model performance also depends on the accuracy, whereby the timing of SGL drainage and the associated lake volume are established. Field investigations have, for example, identified one specific lake-drainage event [2] , which delivered a water volume of 3.6 × 10 6 m 3 at a steady rate between 26 June and 29 June 2010, followed by rapid discharge of 7.4 × 10 6 m 3 on 30 June 2010. The total water volume for that period amounts to 1.1 × 10 7 m 3 , and was originally embedded into our SGL volume loss record of 5.7 × 10 7 m 3 centred on 25 June, with a ±4.5 day of timing uncertainty [10] , generating an average daily velocity at the SHR site of 311 m per year. By correcting the SGL volume loss according to the details given above [2] ( Fig. 2b ), the modelled velocity at the SHR site dropped by ~20%. The high correlation between model and observations ( Table 1 ; Supplementary Table 1 ) suggest that such inaccuracies are overall minor in the record of lake-drainage events. How to cite this article: Bougamont, M. et al. Sensitive response of the Greenland Ice Sheet to surface melt drainage over a soft bed. Nat. Commun. 5:5052 doi: 10.1038/ncomms6052 (2014).